Helicity-dependent three-dimensional optical trapping of chiral microparticles The rule of thumb of tailored optical forces consists in the control of linear momentum exchange between light and matter. This may be done by appropriate selection of the interaction geometry, optical modes or environmental characteristics. Here we reveal that the interplay of the helicity of light and the chirality of matter turns the photon spin angular momentum into an efficient tool for selective trapping of chiral particles. This is demonstrated, both experimentally and theoretically, by exploring the three-dimensional optical trapping of chiral liquid crystal microspheres with circularly polarized Gaussian or Laguerre–Gaussian beams. These results suggest the development of novel optomechanical strategies that rely on the photon helicity towards selective trapping and manipulation of chiral objects by chiral light. Four decades after the first steps in optical trapping and manipulation, optomechanical effects are nowadays widely used for contact-free handling of inert or living entities from nanometric to submillimetric scale. Three-dimensional (3D) optical trapping of an object implies the use of either bell-shaped (that is, Gaussian) or doughnut-shaped (that is, Laguerre–Gaussian) light beams depending on (i) the relationship between the refractive indices of the object and its environment, (ii) the relationship between the object size and the beam waist, and (iii) the spatial structure of the light field itself, see the review papers [1] , [2] , [3] , [4] . Noteworthy, neither the spin angular momentum carried by circularly polarized beams nor the orbital angular momentum carried by Laguerre–Gaussian beams are usually considered as basic ingredients for optical trapping. Indeed, the angular momentum of light has been merely used so far as a tool for addressing the rotational degrees of freedom of optically trapped transparent or absorbing objects, which may be set into spinning and/or orbiting motions [5] , [6] , [7] , [8] , [9] , [10] . Here we show that broken mirror symmetry (that is, chirality) of light–matter interaction can act as an optomechanical trigger for the optical trapping of microparticles. More precisely, we demonstrate the applicability of the photon helicity Λ=±1 (defined as the projection of its spin angular momentum along its propagation direction, in units of ℏ ) for selective optical trapping of transparent microparticles depending on their chirality. The proposed concept is illustrated in Fig. 1 , where a transparent object of chirality χ =±1 (the values correspond to right- and left-handed material, respectively) interacts with an axisymmetric light field. When the given object is located at the point O, the net optical force exerted on it is zero, which refers to an equilibrium position. Helicity-dependent optical trapping implies that the light field exerts, depending on its helicity, either a non-restoring or restoring force on the chiral object displaced from the trapping location O, which in these cases corresponds to either unstable or stable equilibrium, as respectively shown in Fig. 1a,b . In addition, symmetry considerations imply that the phenomenon is invariant under the flipping of both the photon helicity and the material chirality, see Fig. 1c,d . 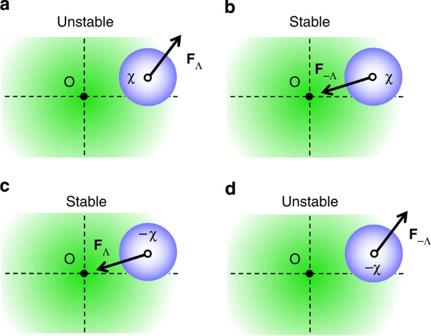Figure 1: Principle of helicity-dependent optical trapping. A chiral object with chiralityχ=±1 is trapped, or not, at the location O, by a light field with helicity Λ=±1. The non-restoring (a,d) or restoring (b,c) nature of the optical forceF, hence the stability of the optical trap, depends on the sign of the product of the helicity of light and the chirality of matter. Figure 1: Principle of helicity-dependent optical trapping. A chiral object with chirality χ =±1 is trapped, or not, at the location O, by a light field with helicity Λ=±1. The non-restoring ( a , d ) or restoring ( b , c ) nature of the optical force F , hence the stability of the optical trap, depends on the sign of the product of the helicity of light and the chirality of matter. Full size image Towards a practical implementation of such an helicity-driven optomechanical behaviour, we use chiral liquid crystal spherical droplets, and our choice is not incidental. Indeed, such prototypical chiral systems have stimulated a significant interest in the context of optical manipulation during the last decade [11] , [12] , [13] and, recently, the idea that the polarization state of light can be used as a control parameter for mechanical actions has emerged. Namely, polarization-controlled attractive–repulsive dynamics [14] , [15] and polarization-controlled optical radiation pressure [16] have been experimentally demonstrated. Then, further studies have respectively led to polarization-dependent angular manipulation in optical tweezers [17] and to the realization of an optofluidic sorter of material chirality driven by chiral light [18] . Although the chirality-sensitive optical trapping remains in its infancy, yet we notice that (i) two-dimensional (2D) trapping has been predicted in a two-beam configuration associated with a light field having mixed helicities [18] and (ii) polarization-dependent 3D trapping in single-beam tweezers has been mentioned in ref. 17 . In this work, we report on a quantitative experimental and theoretical study of 3D optical trapping of chiral liquid crystal microspheres by circularly polarized Gaussian or Laguerre–Gaussian-like laser beams using a two-beam technique. In particular, this allows to consider on-demand selective trapping of chiral particles that satisfy Λ χ =+1, Λ χ =−1 or Λ χ =±1 whatever the particle size, thereby overcoming the stringent limitations associated with the use of single-beam optical tweezers [17] . Indeed, in ref. 17 , chiral particles that satisfy Λ χ =+1 are always trapped, whereas chiral particles satisfying Λ χ =−1 are trapped only for small-enough sizes. In contrast, our results show that all types of chiral particles can be selectively 3D-trapped using an appropriate light field whatever their sizes. Chiral light field Our proposal for helicity-driven selective 3D optical trapping of transparent chiral particles exploits a two-beam technique allowing to trap microparticles at much longer working distances than those accessible to optical tweezers [1] , [2] , [3] , [4] , [5] , [6] , [7] , [8] , [9] , [10] . This technique has been introduced to capture transparent solid glass microspheres by a pair of counterpropagating moderately focused Gaussian beams [19] , [20] . Counterpropagating schemes with high-order optical modes such as Laguerre–Gaussian beams have also been proposed for trapping and manipulation of absorbing particles [21] , [22] . Here we consider both options by using circularly polarized light beams with identical helicity, power and bell- or doughnut-shaped transverse intensity profiles. This is illustrated in Fig. 2a where the set-up is sketched (the upper and lower panels represent simulated spatial intensity distributions). Two continuous-wave laser beams with wavelength λ =532 nm are focused by means of two identical microscope objectives (magnification × 20, numerical aperture 0.4) used in under-filling conditions. This gives the divergence angle measured as θ 0 ≈5° for both beams, hence a beam waist radius w 0 = λ /( πθ 0 )≈2 μm in the focal plane with D ≈500 μm the distance between the two focal planes. 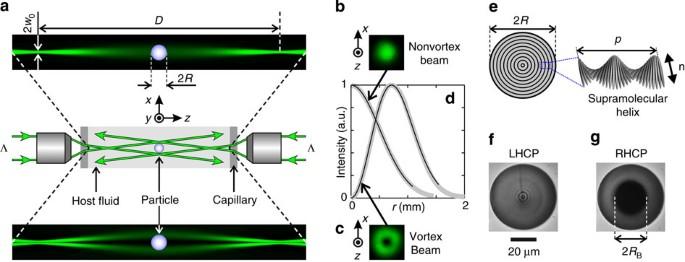Figure 2: Experimental set-up and materials. The set-up consists of two counterpropagating moderately focused non-vortex or vortex beams with identical divergence angle, wavelength, helicity and power.Dis the distance between the two focal planes where beam waist radius isw0. (a) Optical trapping of a transparent spherical chiral liquid crystal droplet of radiusRat the origin (x,y,z)=(0, 0, 0) is considered in all cases, see upper and lower panels. (b–d) Experimental bell- and doughnut-shaped transverse intensity distributions are shown in panelsbandc, whereas their azimuth-averaged radial profiles (thick grey lines in paneld) are described by the fundamental and the first-order Laguerre–Gaussian profiles (thin solid lines in paneld). (e) Sketch of a radial cholesteric droplet. Concentric circles illustrate the onion-like arrangement of the supramolecular pseudo-layers of thicknessp/2 wherepis the helical pitch. (f,g) Full transmission images of a droplet under left/right-handed circularly polarized illumination (LHCP/RHCP) are shown. Figure 2: Experimental set-up and materials. The set-up consists of two counterpropagating moderately focused non-vortex or vortex beams with identical divergence angle, wavelength, helicity and power. D is the distance between the two focal planes where beam waist radius is w 0 . ( a ) Optical trapping of a transparent spherical chiral liquid crystal droplet of radius R at the origin ( x , y , z )=(0, 0, 0) is considered in all cases, see upper and lower panels. ( b – d ) Experimental bell- and doughnut-shaped transverse intensity distributions are shown in panels b and c , whereas their azimuth-averaged radial profiles (thick grey lines in panel d ) are described by the fundamental and the first-order Laguerre–Gaussian profiles (thin solid lines in panel d ). ( e ) Sketch of a radial cholesteric droplet. Concentric circles illustrate the onion-like arrangement of the supramolecular pseudo-layers of thickness p /2 where p is the helical pitch. ( f , g ) Full transmission images of a droplet under left/right-handed circularly polarized illumination (LHCP/RHCP) are shown. Full size image By construction, the light–matter system possesses point symmetry when the particle is located on the beam axis at half the distance between the two focal planes, which defines the origin of the Cartesian coordinate system ( x , y , z ). In practice, we investigate the 3D optical trapping of transparent spherical chiral liquid crystal droplets of radius R located at the origin, where the beam waist radii are w 1 = θ 0 D /2≈20 μm. The non-vortex beams correspond to the output of a single-mode optical fibre used as a spatial filter for the laser light, whereas the vortex beams are obtained by inserting a commercial vortex plate in the path of the beam (see Methods). Experimental bell- and doughnut-shaped transverse intensity profiles are respectively displayed in Fig. 2b,c . These beams can be considered as members of the family of Laguerre–Gaussian modes LG 0l (ref. 23 ), with l the azimuthal index also called the topological charge of the on-axis optical phase singularity carried by the beam. As shown in Fig. 2d , the azimuth-averaged radial intensity profiles of the non-vortex and vortex beams measured at the entrance of the microscope objectives are well described by LG 00 and LG 01 functions, respectively. Chiral material system The material used in this study is a chiral nematic (that is, cholesteric) liquid crystal mesophase. This is a chiral optically anisotropic dielectric medium described by a director n (a unit vector directed along the average local molecular orientation, n and − n being equivalent) that rotates by 2 π around the axis of a supramolecular helix over a distance p called the cholesteric pitch. Such a chiral ordering may be right or left handed. A basic optical property of cholesterics is that the propagation of a plane wave along the helix axis may be forbidden when Λ χ =−1. This is the well-known circular Bragg reflection phenomenon [24] taking place for a certain range of wavelength Δλ= p ( n || − n ⊥ ) centred on λ B = p ( n || + n ⊥ )/2 (ref. 25 ). Here we use the right-handed cholesteric mixture MDA-02-3211 (from Merck) with pitch p =347 nm and average refractive index n =( n || + n ⊥ )/2≈1.6, where n || ≈1.7 and n ⊥ ≈1.5 refer to refractive indices parallel and perpendicular to n at room temperature. In our case, circular Bragg reflection thus occurs for the illumination wavelength λ =532 nm. Spherical chiral microparticles are obtained by dispersing the liquid crystal material in 27 wt% aqueous glycerol solution (this glycerol fraction corresponds to almost isodense emulsion) with refractive index n ext =1.36. The host fluid provides a parallel alignment for the director at the interface of the droplet, hence a radial distribution of the helix axes. By doing so, we obtain onion-like structured droplets with R >> p (ref. 26 ), as sketched in Fig. 2e . Practically, such droplets have two key advantages. Indeed (i) their spherical symmetry prevents from any droplet orientation issue, hence facilitating the modelling task (as a matter of fact, the symmetry is broken by the radial defect that is required for topological reasons to close the structure [27] ; however, no influence of the defect on the reported phenomena has been detected) and (ii) their optical scattering properties strongly depend on the photon helicity due to the circular Bragg reflection phenomenon, which gives rise to helicity-dependent optical forces [16] . The latter point is illustrated in Fig. 2f,g that display full transmission images of a radial cholesteric droplet under left-handed (Λ=+1) and right-handed (Λ=−1) circularly polarized illumination at 532 nm wavelength, respectively. The zero-transmission circular area of radius R B in Fig. 2g is associated with the circular Bragg photonic bandgap and indicates that the droplet behaves as a perfect spherical mirror with radius of curvature R and cross-section radius R B . Noticeably, the half-apex angle θ B,ext =arcsin( R B / R ) of the corresponding Bragg cone does not depend on the droplet radius and is related to the intrinsic angle θ B through the Snell–Descartes relationship n ext sin θ B,ext = n sin θ B , with θ B ≈25° for the chosen material [16] . Model Following our experimental framework, the description of optical 3D trapping of onion-like cholesteric droplets with chirality χ is handled by considering the interaction between two paraxial counterpropagating Laguerre–Gaussian beams LG 0l and a non-deformable transparent sphere of radius R endowed with helicity-dependent light scattering properties and immersed in a lossless viscous fluid with refractive index n ext and dynamical viscosity η . More precisely, within a ray-optics approach whose relevance is ensured by λ ≪ R , the particle is modelled as a perfect spherical mirror when the two following conditions are fulfilled: (i) Λ χ =−1 and (ii) the angle between an incident ray and the normal to the sphere at the hitting point is smaller than θ B,ext . Otherwise, the particle is described as a uniform dielectric sphere of refractive index n . In the general case of a droplet whose centre of mass is located at ( x , y , z )=( r cos ϕ , r sin ϕ , z ), the optical force exerted on it is retrieved from the first principle of mechanics by evaluating the balance of linear momentum. Following the approach detailed in the Methods section, we calculate a total optical force of the form F = F r ( r , z ) u r + F z ( r , z ) u z , where ( u r , u ϕ , u z ) refers to the orthonormal Cartesian coordinate basis ( u x , u y , u z ) rotated by an angle ϕ around the z axis. Note that the invariance with respect the azimuthal angle ϕ results from the fact that the two beams are coaxial and have axisymmetric intensity distributions. Simulations Owing to the symmetry of the light–matter system, the optical force exerted on the droplet vanishes at the origin ( r =0, z =0) whatever are the values of the parameters. In weightless conditions, which is roughly the case in our experiments, the origin thus corresponds to the point where the droplet may be optically trapped in 3D. This occurs if both conditions ∂ F z /∂ z <0 and ∂ F r /∂ r <0 are fulfilled. These conditions are numerically investigated for non-vortex (l=0) and vortex (l≠0) beams with Λ χ =±1 and variable geometrical parameters θ 0 and w 1 / R . The results for l=0, 1, 2 and 3 are summarized in Fig. 3a–d , where the existence criterion of 3D trapping in the plane of parameters ( w 1 / R , θ 0 ) is identified as coloured areas. In addition, the role played by the photon helicity is emphasized by the distinction made between 3D trapping for Λ χ =+1 alone, Λ χ =−1 alone and Λ χ =±1 simultaneously. 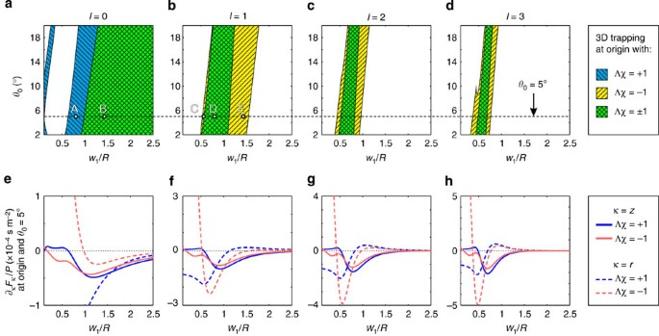Figure 3: Helicity-dependent 3D optical trapping simulations. (a–d) Existence of 3D trapping in the plane of parameters (w1/R,θ0) depending on the photon helicity forw1=20 μm and l=0, 1, 2 and 3, where the material parameter values are those of our experiments. Three different coloured/hatched regions refer to trapping existence for the cases Λχ=+1 alone, Λχ=−1 alone and Λχ=±1 simultaneously. Letters A, B, C, D and E correspond to the valuesw1/R≈0.8, 1.43, 0.59, 0.74 and 1.43. (e–h) Partial derivatives of the optical force components at origin per unit power for a beam divergence angleθ0=5°. Figure 3: Helicity-dependent 3D optical trapping simulations. ( a – d ) Existence of 3D trapping in the plane of parameters ( w 1 / R , θ 0 ) depending on the photon helicity for w 1 =20 μm and l=0, 1, 2 and 3, where the material parameter values are those of our experiments. Three different coloured/hatched regions refer to trapping existence for the cases Λ χ =+1 alone, Λ χ =−1 alone and Λ χ =±1 simultaneously. Letters A, B, C, D and E correspond to the values w 1 / R ≈0.8, 1.43, 0.59, 0.74 and 1.43. ( e – h ) Partial derivatives of the optical force components at origin per unit power for a beam divergence angle θ 0 =5°. Full size image It appears from simulations that 3D trapping under Λ χ =−1, as is the case for chiral particles exhibiting Bragg reflection of light, or Λ χ =+1, when our chiral particles are described as non-chiral dielectric spheres, may be allowed whatever is l depending on the used parameters. The trapping existence region, however, tends to reduce as l increases, as shown in Fig. 3a–d . Moreover, when 3D trapping is expected to occur simultaneously for Λ χ =±1, we note that there is a significant dependence of the trap features on the photon helicity. Indeed, the longitudinal (along z ) and transverse (perpendicular to z ) stiffness of the optical trap both depend on Λ χ . This is illustrated in Fig. 3e–h , where the partial derivatives of the optical force components per unit power, ∂ κ F κ / P with ∂ κ (·)≡ ∂(·)/∂ κ and κ =( r , z ), are shown for θ 0 =5°, which corresponds to the beam divergence used in the experiments. Experimental validation of the model In practice, the demonstration of helicity-dependent 3D optical trapping is achieved by studying the behaviour of onion-like liquid crystal droplets irradiated by two Gaussian or Laguerre–Gaussian beams under the geometry specified in the experimental approach description. The demonstration consists in testing whether the beams can trap a droplet of radius R at the origin and, if the trapping is achieved, in the observation of the droplet behaviour after the helicity is flipped from Λ to −Λ. Qualitative comparison between experiments and simulations is summarized in Fig. 4 where the upper row displays initial trapping situations for cases A, B, C, D and E, see Fig. 3a–d , which are representative of all possible predicted situations for l=0 and 1. Then, flipping the helicity of the beams from Λ to −Λ, we observe that the droplet is no longer trapped in cases A, C and E, whereas it remains trapped at origin in cases B and D. All these observations agree with theoretical expectations, thereby validating the main features of the optical force field at the origin. 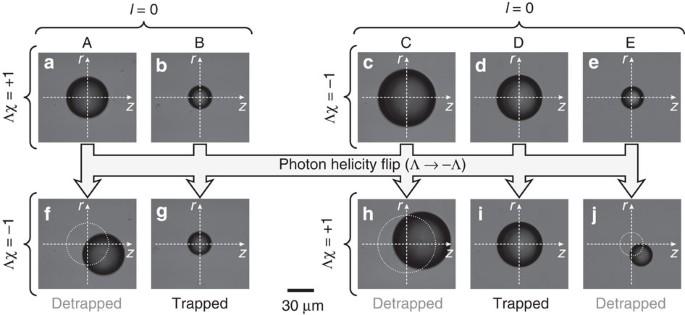Figure 4: Helicity-dependent 3D optical trapping observations. (a–e) Snapshots of onion-like chiral liquid crystal droplets optically trapped at origin under powerP≈50 mW in situations tagged by the letters A, B, C, D and E inFig. 3a–e, which, respectively, correspond tow1/R≈0.8, 1.43, 0.59, 0.74 and 1.43. Situations A and B refer to Gaussian beams with Λχ=+1 (a,b), whereas C, D and E refer to first-order Laguerre–Gaussian beams with Λχ=−1 (c–e). For l=0, helicity flip leads to detrapping of the larger droplet (f), whereas the smaller one is kept trapped at the origin (g). For l=1, helicity flip leads to detrapping for both the larger and the smaller droplets (h,j), whereas the droplet with intermediate size remains trapped at the origin (i). Figure 4: Helicity-dependent 3D optical trapping observations. ( a – e ) Snapshots of onion-like chiral liquid crystal droplets optically trapped at origin under power P ≈50 mW in situations tagged by the letters A, B, C, D and E in Fig. 3a–e , which, respectively, correspond to w 1 / R ≈0.8, 1.43, 0.59, 0.74 and 1.43. Situations A and B refer to Gaussian beams with Λ χ =+1 ( a , b ), whereas C, D and E refer to first-order Laguerre–Gaussian beams with Λ χ =−1 ( c – e ). For l=0, helicity flip leads to detrapping of the larger droplet ( f ), whereas the smaller one is kept trapped at the origin ( g ). For l=1, helicity flip leads to detrapping for both the larger and the smaller droplets ( h , j ), whereas the droplet with intermediate size remains trapped at the origin ( i ). Full size image Force field quantitative analysis Since our model has been derived in a general framework, the net optical force exerted on the droplet can be evaluated for any location ( r , z ). This is illustrated in Fig. 5a,b for two representative cases that lead to stable 3D trapping at the origin, namely {l=0, Λ χ =+1, w 1 / R =2/3} and {l=1, Λ χ =−1, w 1 / R =1}, with θ 0 =5° and w 1 =20 μm. The latter situations actually correspond to cases A and D in Fig. 3 . In Fig. 5a,b , arrows indicate the direction of the optical force, whereas colour maps refer to the force magnitude. That said, we note that the setting up of a quantitative assessment may benefit from the symmetries of the light–matter system, which imply F r (0, z )=0 and F z ( r , 0)=0. Indeed, this allows the independent study of (i) the axial force F z along the z axis and (ii) the radial force F r in a direction perpendicular to z passing through the origin. 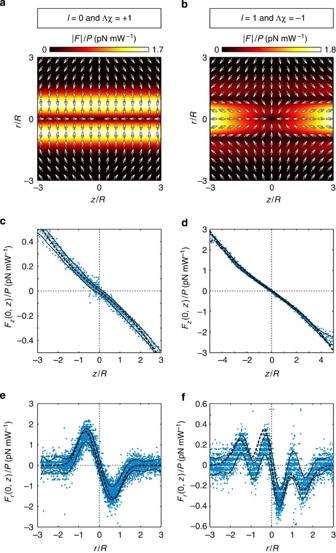Figure 5: Quantitative analysis of 3D optical force fields. (a,b) Spatial distribution of the magnitude (colour map) and orientation (vector plot) of the calculated optical force exerted on a droplet located around the origin, namely −3R<z<3Rand −3R<r<3R, for {l=0, Λχ=+1,w1/R=2/3} and {l=1, Λχ=−1,w1/R=1}, withθ0=5° andw1=20 μm. (c,d) Experimental data for the longitudinal component of the force along thezaxis,Fz(0,z). (e,f) Experimental data for the transverse component of the force along the axisrthat passes through the origin,Fr(r, 0). Experimental conditions: the experimental data set (dot markers) corresponds to 40 independent realizations, whose standard deviation range is indicated by solid curves, whereas dashed curves are the results of simulations without adjustable parameters. Left panels correspond toP≈20 mW andR=29 μm, whereas right panels refer toP≈70 mW andR=20 μm. The constant drag velocity for radial force measurements isV0=36 μm s−1, see text for details. Figure 5: Quantitative analysis of 3D optical force fields. ( a , b ) Spatial distribution of the magnitude (colour map) and orientation (vector plot) of the calculated optical force exerted on a droplet located around the origin, namely −3 R < z <3 R and −3 R < r <3 R , for {l=0, Λ χ =+1, w 1 / R =2/3} and {l=1, Λ χ =−1, w 1 / R =1}, with θ 0 =5° and w 1 =20 μm. ( c , d ) Experimental data for the longitudinal component of the force along the z axis, F z (0, z ). ( e , f ) Experimental data for the transverse component of the force along the axis r that passes through the origin, F r ( r , 0). Experimental conditions: the experimental data set (dot markers) corresponds to 40 independent realizations, whose standard deviation range is indicated by solid curves, whereas dashed curves are the results of simulations without adjustable parameters. Left panels correspond to P ≈20 mW and R =29 μm, whereas right panels refer to P ≈70 mW and R =20 μm. The constant drag velocity for radial force measurements is V 0 =36 μm s −1 , see text for details. Full size image In practice, the net optical force field is retrieved by recording the motion of the droplet. In the limit of small Reynolds number, as is the case in our experiments, the expression for the light-induced droplet velocity is obtained from the balance between the viscous force exerted by the surrounding fluid on the moving droplet and the driving optical force. Namely F κ ( r , z )=6 πηRε κ ( r , z ) with η =2 mPa s. In addition, we apply different strategies for the measurements of F z and F r . On one hand, concerning F z , a droplet initially trapped at the origin is optically displaced along z by turning off one of the two beams. When being restored, the optical field guides the droplet back to the origin where it is trapped again. The recorded droplet motion gives access to the dependence of ε z on z , hence to F z (0, z ). The reverse procedure then completes the analysis. On the other hand, motivated by the fact that there is no all-optical way to displace at will the droplet in a direction perpendicular to z , we use an alternative approach to measure F r ( r , 0). It consists in using a droplet as an optomechanical probe in order to map the force field. Namely, the capillary is dragged at a constant velocity V 0 along r so that the immersed droplet moves in a direction perpendicular to z passing through the origin. The recorded motion of the droplet thus gives the net velocity V r ( r , 0)= V 0 + ε r ( r , 0), from which we extract F r ( r , 0)=6 πηRε r ( r , 0). Following the above protocols, data have been collected for 40 independent realizations. The results for F z (0, z ) are shown in Fig. 5c,d for l=0 and 1, whereas those for F r ( r , 0) are shown in Fig. 5e,f for l=0 and 1, see dot markers. Recalling that there is no adjustable parameters in our model, the comparison with simulations (dashed curves) gives a satisfying agreement with the data, whose standard deviation range is indicated by solid curves. The fact that a weightless model quantitatively describes experimental data emphasizes the choice of a quasi-isodense host fluid environment. However, we stress that such a framework has been merely chosen to ease the practical implementation rather than being a necessary condition to observe helicity-dependent 3D optical trapping. To prove it, we have calculated the equilibrium position of the droplet for the two situations presented in Fig. 5 but accounting for a mismatch between the density of the particle, ρ part and that of the external fluid, ρ ext . The gravitational acceleration is taken along x as is the case in practice. The results are presented in Fig. 6 where the dependence of the magnitude of the x coordinate of the equilibrium positions ( x eq , 0) is shown as a function of the density mismatch |Δ ρ |=| ρ part − ρ ext | per unit power. Solid curves refer to 3D optical trapping whereas dotted ones correspond to 2D trapping, the equilibrium position being unstable in the z direction. Above analysis emphasizes that chiral particles exhibiting Bragg reflection of light can be easily trapped in 3D by contra-propagating vortex beams over a wide range of |Δ ρ |. For instance, a pair of LG 01 beams with P =1 W should trap a sphere with density up to 1.3 g cm −3 in the air. This might be explored by using solidified radial cholesteric microspheres [14] instead of liquid ones. In contrast, the Gaussian beam trapping of particles that do not exhibit Bragg reflection is characterized with more stringent density mismatch restrictions. Indeed, for l=0 and present beam parameters, 3D optical trapping occurs if |Δ ρ |/ P <0.04 g cm −3 W −1 . Such a condition is here easily fulfilled since the host fluid density can be tuned with 10 −3 g cm −3 accuracy by adjusting the glycerol concentration. 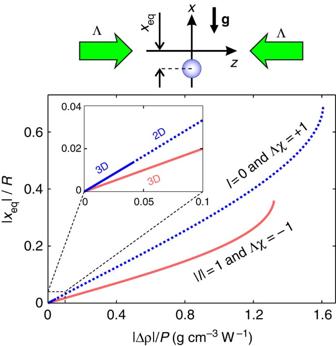Figure 6: Role of gravity. Simulated equilibrium positionxeqof a chiral microparticle irradiated by two counterpropagating beams as a function of density mismatch between the particle and the host medium. Optical and material parameters are those used in the experiments, except the droplet density that is taken here as the variable quantity. Upper sketch:gis the gravitational acceleration. Plot: solid curves correspond to 3D optical trapping whereas dotted ones refer to 2D trapping of the particle in the (z=0) plane and unstable trapping alongz. Figure 6: Role of gravity. Simulated equilibrium position x eq of a chiral microparticle irradiated by two counterpropagating beams as a function of density mismatch between the particle and the host medium. Optical and material parameters are those used in the experiments, except the droplet density that is taken here as the variable quantity. Upper sketch: g is the gravitational acceleration. Plot: solid curves correspond to 3D optical trapping whereas dotted ones refer to 2D trapping of the particle in the (z=0) plane and unstable trapping along z . Full size image Another issue concerns the possible actuation of the rotational degree of freedom of the trapped microparticles. Indeed, both trapping beams may carry spin and orbital angular momentum depending on the chosen configuration. However, we note that our experiments deal with counterpropagating beams with identical geometrical parameters, helicity and power. This prevents from any net deposition of spin angular momentum since any contribution of one beam is balanced by the contribution of the second beam, although each beam independently deposits spin angular momentum when circular Bragg reflection takes place. Regarding the transfer of orbital angular momentum from light to matter, it vanishes when the droplet lies on the beam axes by virtue of axisymmetry (which implies the radial defect to be aligned on the beam axis). Consistently, we found no experimental indication of neither spinning nor orbiting motion for all studied trapping events. To conclude, we demonstrated both experimentally and theoretically that the photon helicity can be used as a trigger to optically trap, in three dimensions and in a selective manner, chiral particles with non-chiral morphology. The driving mechanism consists in actuation of the material translational degrees of freedom by the intrinsic rotational ones of light. Present concept, whose demonstration addresses the case of spherical chiral particles, might be extended to non-chiral objects endowed with chiral morphology by using orbital angular momentum instead of spin angular momentum of light as a control parameter. To this aim, the orbital counterpart of the circular Bragg reflection phenomenon might be worth considering, see ref. 28 and references therein. Although present results concern a given chiral material system explored at the 1–100 μm scale, combining this first experimental step to several recent theoretical studies on helicity-dependent optomechanics at the submicrometre scale [29] , [30] , [31] , [32] should motivate the development of practical realization of optomechanical strategies for selective optical trapping and manipulation of chiral objects whose application potential is multidisciplinary by nature. Preparation of the vortex beams Optical vortices are experimentally obtained by using a radial polarization converter (Altechna R&D) illuminated by a circularly polarized collimated Gaussian beam. The output light field is contra-circularly polarized with respect to the input polarization state, and possesses on-axis phase singularity with topological charge l=±1 (the sign depends on the input polarization state handedness). As shown in Fig. 2c,d , one obtains a vortex beam having an LG 01 -like transverse intensity distribution. Helicity control Fast remote flipping of the photon helicity in the optical system was essential for the experiments reported in Fig. 4 . The required control is achieved via two identical electrically addressed liquid crystal variable retarders (Meadowlark Optics, Inc.) placed in the path of each of the two beams. Derivation of the model The first step towards the determination of the net optical force exerted on the chiral sphere is to evaluate the contribution d F due to the incident light impinging on the surface element d S ( θ , φ )= R 2 sin θ d θ d φ with ( θ , φ ) the polar and azimuthal angles in the spherical coordinate system originating at the droplet centre, see Fig. 7 . In the present case, 0≤ θ ≤ π /2 and π /2≤ θ ≤ π thus correspond to the beam propagating towards z <0 and z >0, respectively. 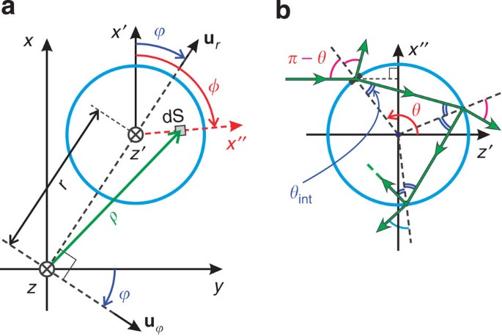Figure 7: Definitions and notations. (a,b) Ray tracing and definitions used in the model developed to describe the helicity-dependent net optical force exerted on a droplet. Figure 7: Definitions and notations. ( a , b ) Ray tracing and definitions used in the model developed to describe the helicity-dependent net optical force exerted on a droplet. Full size image To calculate the net change of linear momentum of the light field as it is scattered by the droplet within the ray-optics approach, we attribute the Minkowski linear momentum ℏ k per photon pointing along each geometrical ray, with ℏ the reduced Planck constant and k the wavevector. For a droplet whose centre of mass is located at ( x , y , z )=( r cos ϕ , r sin ϕ , z ), one thus gets where c is the speed of light in vacuum, ( u r , u ϕ , u z ) refers to the orthonormal Cartesian coordinate basis ( u x , u y , u z ) rotated by an angle φ around the z axis, and is the spatial intensity distribution of a LG 0l beam, with ξ the distance from its focal plane and ρ the distance from its axis, P its total power, , w 0 the beam waist and the Rayleigh range. In addition, we have with sgn the sign function. Moreover, f ⊥ ( θ ) and f || (θ) characterize how the ‘energy of an incident ray’ is apportioned between the reflected, refracted and scattered rays that originate from the incident ray. On one hand, for non-Bragg rays (that is, rays that are not totally reflected by the droplet), we get [33] where and =1− are the reflectance and transmittance of the droplet interface, with θ int =sgn(cos θ ) arcsin[( n ext / n ) sin θ ] the signed angle of refraction. Accounting for the incident circular polarization state and discarding the polarization projection on the local frame of incidence, we also assume that ( θ )=[ || ( θ )+ ⊥ ( θ )]/2 with || ( θ )=[tan( θ − θ int )/tan( θ + θ int )] 2 and ⊥ ( θ )=[sin( θ − θ int )/sin( θ + θ int )] 2 the reflectance coefficients of plane waves polarized parallel and perpendicular to the incidence plane [34] . On the other hand, one straightforwardly gets for Bragg rays (that is, rays that are totally reflected by the droplet) The total force F = F r u r + F ϕ u ϕ + F z u z exerted on the droplet is obtained by integrating the elementary force over the sphere: Noticeably, the above equations lead to ∂ F r /∂ ϕ =0 and ∂ F z /∂ ϕ =0, as expected from coaxial light beams having axisymmetric intensity distributions. The net optical force exerted on the droplet is thus written How to cite this article: Tkachenko, G. and Brasselet, E. Helicity-dependent three-dimensional optical trapping of chiral microparticles. Nat. Commun. 5:4491 doi: 10.1038/ncomms5491 (2014).